ALKBH8-mediated formation of a novel diastereomeric pair of wobble nucleosides in mammalian tRNA Mammals have nine different homologues (ALKBH1–9) of the Escherichia coli DNA repair demethylase AlkB. ALKBH2 is a genuine DNA repair enzyme, but the in vivo function of the other ALKBH proteins has remained elusive. It was recently shown that ALKBH8 contains an additional transfer RNA (tRNA) methyltransferase domain, which generates the wobble nucleoside 5-methoxycarbonylmethyluridine (mcm 5 U) from its precursor 5-carboxymethyluridine (cm 5 U). In this study, we report that ( R )- and ( S )-5-methoxycarbonylhydroxymethyluridine (mchm 5 U), hydroxylated forms of mcm 5 U, are present in mammalian , and , respectively, representing the first example of a diastereomeric pair of modified RNA nucleosides. Through in vitro and in vivo studies, we show that both diastereomers of mchm 5 U are generated from mcm 5 U, and that the AlkB domain of ALKBH8 specifically hydroxylates mcm 5 U into ( S )-mchm 5 U in . These findings expand the function of the ALKBH oxygenases beyond nucleic acid repair and increase the current knowledge on mammalian wobble uridine modifications and their biogenesis. Transfer RNA (tRNA) modification is important both for correct folding and for optimal interaction with components of the protein synthesis machinery, such as aminoacyl transferases, messenger RNA (mRNA) and the ribosome. The nucleotide at the wobble position in the anticodon loop of tRNA interacts with the third nucleotide of the codon in mRNA, and wobble uridines are usually modified, both in bacteria and eukaryotes [1] , [2] . Modification of wobble uridines ensures efficient decoding of both cognate and non-cognate codons [3] , [4] , and prevents misreading of codons from 'split' boxes, where purine- and pyrimidine-ending codons encode different amino acids [1] . In eukaryotes, most wobble uridines carry the modification 5-methoxycarbonylmethyluridine (mcm 5 U), 5-carbamoylmethyluridine (ncm 5 U) or derivatives thereof ( Fig. 1a ). These modifications and their biogenesis have been most closely studied in the yeast Saccharomyces cerevisiae . Here, tRNA isoacceptors that contain ncm 5 U decode in the 'family' codon boxes, in which all four codons encode the same amino acid, whereas tRNAs containing mcm 5 U usually decode in the split codon boxes. The Elongator complex has been shown to mediate an early step in mcm 5 U/ncm 5 U formation [5] , whereas the final methyl esterification reaction leading to the formation of mcm 5 U is catalysed by the methyltransferase (MT) Trm9 (ref. 6 ). 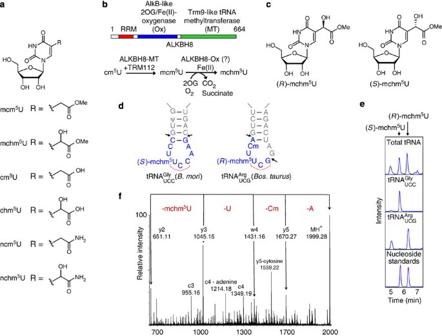Figure 1: Presence of two mchm5U diastereomers in the wobble position of mammalian tRNA. (a) Wobble uridine modifications described in the present work. mcm5U, 5-methoxycarbonylmethyluridine; mchm5U, 5-methoxycarbonylhydroxymethyluridine; chm5U, 5-carboxyhydroxymethyluridine; cm5U, 5-carboxymethyluridine; ncm5U, 5-carbamoylmethyluridine; nchm5U, 5-carbamoylhydroxymethyluridine. (b) Domain structure and proposed function of ALKBH8. RRM, RNA recognition motif. Together with the accessory protein TRM112, the MT domain of ALKBH8 converts cm5U into mcm5U. In the present work, the ALKBH8 oxygenase has been investigated for its ability to hydroxylate mcm5U into mchm5U. (c) Chemical structure of the two mchm5U diastereomers. (d) The anticodon stem-loop region of silkwormand calf. Anticodon (red line) containing products (blue) generated by RNase T1 cleavage (arrows), and analysed by MALDI-TOF MS, are indicated. (e) LC–MS/MS analysis of mchm5U nucleosides in calf liver total tRNA and isolated isoacceptors. (f) MALDI-quadrupole TOF tandem mass spectrometry of the RNase T1 product harbouring the anticodon of. Fragmentation pattern suggests the sequence A-Cm-U-mchm5U-C-G>p as indicated. c-Ions contain the original 5′-end after cleavage of the phophodiester bond between the phosphorous and the 5′-oxygen; y-ions contain the original 3′-end after cleavage of the phophodiester bond between the phosphorous and the 5′-oxygen. w-Ions contain the original 3′-end after cleavage of the phophodiester bond between the 3′-carbon and the 3′-oxygen. The associated number gives the size of the fragment ion in nucleotide residues. >p denotes 2′–3′ cyclic phosphate. Figure 1: Presence of two mchm 5 U diastereomers in the wobble position of mammalian tRNA. ( a ) Wobble uridine modifications described in the present work. mcm 5 U, 5-methoxycarbonylmethyluridine; mchm 5 U, 5-methoxycarbonylhydroxymethyluridine; chm 5 U, 5-carboxyhydroxymethyluridine; cm 5 U, 5-carboxymethyluridine; ncm 5 U, 5-carbamoylmethyluridine; nchm 5 U, 5-carbamoylhydroxymethyluridine. ( b ) Domain structure and proposed function of ALKBH8. RRM, RNA recognition motif. Together with the accessory protein TRM112, the MT domain of ALKBH8 converts cm 5 U into mcm 5 U. In the present work, the ALKBH8 oxygenase has been investigated for its ability to hydroxylate mcm 5 U into mchm 5 U. ( c ) Chemical structure of the two mchm 5 U diastereomers. ( d ) The anticodon stem-loop region of silkworm and calf . Anticodon (red line) containing products (blue) generated by RNase T1 cleavage (arrows), and analysed by MALDI-TOF MS, are indicated. ( e ) LC–MS/MS analysis of mchm 5 U nucleosides in calf liver total tRNA and isolated isoacceptors. ( f ) MALDI-quadrupole TOF tandem mass spectrometry of the RNase T1 product harbouring the anticodon of . Fragmentation pattern suggests the sequence A-Cm-U-mchm 5 U-C-G>p as indicated. c-Ions contain the original 5′-end after cleavage of the phophodiester bond between the phosphorous and the 5′-oxygen; y-ions contain the original 3′-end after cleavage of the phophodiester bond between the phosphorous and the 5′-oxygen. w-Ions contain the original 3′-end after cleavage of the phophodiester bond between the 3′-carbon and the 3′-oxygen. The associated number gives the size of the fragment ion in nucleotide residues. >p denotes 2′–3′ cyclic phosphate. Full size image The 2OG/Fe(II) (2-oxoglutarate- and Fe 2+ -dependent) oxygenase superfamily encompasses enzymes involved in important processes, for example, generation of hydroxyproline in collagen, regulation of hypoxia-responsive genes, demethylation of histone proteins, nucleic acid repair and, as discovered recently, introduction of the epigenetic modification 5-hydroxymethylcytosine (5hmC) in DNA [7] , [8] , [9] . The 2OG/Fe(II) oxygenase AlkB from Escherichia coli is a repair enzyme that can demethylate lesions in DNA and RNA, such as 1-methyladenine and 3-methylcytosine [10] , [11] , [12] . Bioinformatics analysis has identified a family of nine different mammalian AlkB homologues (ALKBH), including the obesity-associated protein FTO [13] , [14] . Although in vitro repair activities have been observed for some ALKBH proteins [10] , [13] , [15] , [16] , only ALKBH2 has been firmly established as a repair enzyme [17] , and non-repair functions have also been proposed [18] , [19] , [20] . We and others recently showed that ALKBH8 contains a MT domain, which is the functional mammalian Trm9 homologue, and requires a small accessory protein, TRM112, for activity ( Fig. 1b ) [21] , [22] . As hydroxylation is the primary reaction catalysed by 2OG/Fe(II) oxygenases in animals, and as the MT domain of ALKBH8 is involved in mcm 5 U biogenesis, we were intrigued by a report documenting the presence of 5-methoxycarbonylhydroxymethyluridine (( S )-mchm 5 U), a hydroxylated form of mcm 5 U, in from the silkworm Bombyx mori [23] ( Fig. 1c,d ). Mammalian and worm are highly similar, and the primary sequence of the anticodon loop is identical ( Supplementary Fig. S1 ). This suggested that ( S )-mchm 5 U may be present also in mammalian tRNA, and that the ALKBH8 oxygenase could be responsible for its formation ( Fig. 1b ). Indeed, whilst our manuscript was under preparation, Fu et al . independently reported that the AlkB domain of murine ALKBH8 can hydroxylate wobble mcm 5 U into ( S )-mchm 5 U in a synthetic substrate resembling the anticodon stem-loop of [24] . In the present work, we demonstrate that ( S )-mchm 5 U is found in the wobble position of mammalian , and that its diastereomer, ( R )-mchm 5 U, is found in . Moreover, we show through studies of gene-targeted mice and recombinant enzymes that the MT domain of ALKBH8 provides the mcm 5 U precursor required for formation of mchm 5 U in and , whereas its AlkB domain represents an evolutionary conserved oxygenase that catalyses the hydroxylation of wobble mcm 5 U to ( S )-mchm 5 U in . Analysis of mchm 5 U modifications in mammalian tRNA To investigate the possible presence of mchm 5 U in mammalian tRNA, we analysed the modification status of nucleosides from bovine tRNA by liquid chromatography coupled to tandem mass spectrometry (LC–MS/MS). In this analysis, a triple-quadrupole mass spectrometer was used to specifically select the relevant nucleoside ions, induce fragmentation and detect the resulting nucleobase fragment ions. Additional specificity was obtained by comparing chromatographic retention times with those of synthetic nucleoside standards. This allows highly specific, sensitive and simultaneous quantification of several nucleosides. Intriguingly, substantial amounts of both the S and R diastereomers of mchm 5 U were detected in total bovine tRNA nucleosides ( Fig. 1e ). We next isolated individual, wobble uridine-containing isoacceptors by hybridization to complementary, immobilized DNA oligonucleotides. We found, as expected, ( S )-mchm 5 U to be present in , whereas contained ( R )-mchm 5 U ( Fig. 1e ). We were unable to identify additional wobble uridine-containing tRNA isoacceptors carrying a mchm 5 U modification (data not shown). The presence of wobble ( R )-mchm 5 U in was supported by matrix-assisted laser desorption/ionization (MALDI)-time-of-flight (TOF) mass spectrometry of an RNase T1 digest of the purified isoacceptor. Sequencing by MALDI-quadrupole-TOF tandem mass spectrometry confirmed the presence of mchm 5 U at the wobble position, and the fragmentation pattern also revealed ribose methylation of C32 (ref. 25 ), a very common tRNA modification ( Fig. 1d,f ) [2] . Analysis of wobble uridines in Alkbh8-targeted mice To address the possible role of the ALKBH8 oxygenase in mchm 5 U biogenesis, we used a mouse model, in which essential exons of the Alkbh8 gene had been deleted ( Alkbh8 −/− ; ref. 22 ). Moreover, we developed two novel 'knock-in' (KI) mice in which an oxygenase-deficient Alkbh8 transgene ( KI(MT + )) or a MT-deficient Alkbh8 transgene ( KI(Ox + )) was expressed from the Rosa26 or Hprt loci, respectively ( Supplementary Figs S2–S5 ). These transgenes, or the combination of the two ( KI ( MT + /Ox + )), were introduced into the Alkbh8 −/− background ( Fig. 2a ). The expression of the transgenes was verified by reverse transcription and PCR (data not shown). All the mouse models were devoid of any obvious phenotype. First, we analysed by LC–MS/MS, total tRNA nucleosides from the different mice for the presence of the two mchm 5 U diastereomers. As expected, wild-type (WT) tRNA contained both ( R )- and ( S )-mchm 5 U ( Fig. 2b ). tRNA from the Alkbh8 −/− and KI(Ox + ) mice, which lack functional MT activity, were devoid of both ( R )- and ( S )-mchm 5 U, whereas the KI(MT + ) tRNA contained exclusively ( R )-mchm 5 U. These data indicate that the formation of either mchm 5 U diastereomer requires the MT function, whereas the oxygenase is required for the formation of ( S )-mchm 5 U only. This implies that a second unknown oxygenase, in the following referred to as OxX, is responsible for the hydroxylation of mcm 5 U to ( R )-mchm 5 U. Furthermore, KI(MT + /Ox + ) tRNA contained, like WT tRNA, both mchm 5 U stereoisomers ( Fig. 2b ), indicating that the MT and oxygenase activities of ALKBH8 can be uncoupled and provided by two individual proteins. 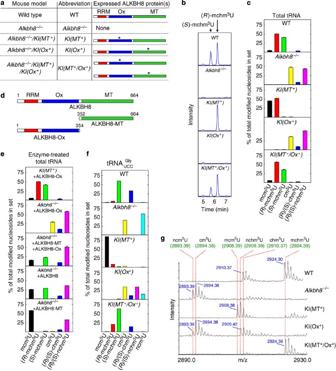Figure 2: Modification status of tRNA from Alkbh8-targeted mice. (a) Schematic representation of the ALKBH8 proteins expressed in the different mouse models. An asterisk indicates that the domain has been inactivated by point mutations. (b) Analysis ofRandSdiastereomers of mchm5U in total tRNA from gene-targeted mice. Murine tRNA was enzymatically degraded to nucleosides, which were analysed by LC–MS/MS. (c) Quantification of uridine modifications in total murine tRNA by LC–MS/MS. The level of each nucleoside is expressed as the molar percentage of the total amount of the modifications indicated in the figure. (d) Recombinant,E. coli-expressed ALKBH8 proteins, or individual domains, used for incubation with murine tRNA. (e) Modification status of murine tRNA treated with human ALKBH8 or its individual domains. ALKBH8 and ALKBH8-MT were associated with co-expressed, co-purified TRM112. (f) Modification status of murinemeasured by LC–MS/MS. (g) MALDI-TOF analysis of the anticodon-containing RNase T1 product of. The theoretical monoisotopic mass (green) as well as the measured mass (blue) of relevant modifications are indicated. Because of the natural isotope distribution, each modification gives rise to a cluster of peaks with 1.0 Da spacing where the leftmost peak corresponds to the monoisotopic mass. Overlapping isotope clusters from ncm5U and cm5U with clearly distorted peak patterns occur in theAlkbh8−/−andKI(Ox+) samples. Error bars represent range between duplicate samples in a typical experiment. Figure 2: Modification status of tRNA from Alkbh8-targeted mice. ( a ) Schematic representation of the ALKBH8 proteins expressed in the different mouse models. An asterisk indicates that the domain has been inactivated by point mutations. ( b ) Analysis of R and S diastereomers of mchm 5 U in total tRNA from gene-targeted mice. Murine tRNA was enzymatically degraded to nucleosides, which were analysed by LC–MS/MS. ( c ) Quantification of uridine modifications in total murine tRNA by LC–MS/MS. The level of each nucleoside is expressed as the molar percentage of the total amount of the modifications indicated in the figure. ( d ) Recombinant, E. coli -expressed ALKBH8 proteins, or individual domains, used for incubation with murine tRNA. ( e ) Modification status of murine tRNA treated with human ALKBH8 or its individual domains. ALKBH8 and ALKBH8-MT were associated with co-expressed, co-purified TRM112. ( f ) Modification status of murine measured by LC–MS/MS. ( g ) MALDI-TOF analysis of the anticodon-containing RNase T1 product of . The theoretical monoisotopic mass (green) as well as the measured mass (blue) of relevant modifications are indicated. Because of the natural isotope distribution, each modification gives rise to a cluster of peaks with 1.0 Da spacing where the leftmost peak corresponds to the monoisotopic mass. Overlapping isotope clusters from ncm 5 U and cm 5 U with clearly distorted peak patterns occur in the Alkbh8 −/− and KI(Ox + ) samples. Error bars represent range between duplicate samples in a typical experiment. Full size image To study how manipulation of ALKBH8 activity affects the formation of modified uridines in vivo , we also measured the levels of various other modifications ( Fig. 2c , Supplementary Figs S6 and S7 ). tRNA isolated from KI(MT + ) mice displayed a strong accumulation of mcm 5 U, consistent with mcm 5 U being a direct substrate for the ALKBH8 oxygenase. In agreement with previous results [22] , we detected substantial amounts of 5-carboxymethyluridine (cm 5 U) and elevated levels of ncm 5 U in tRNA from the MT-deficient Alkbh8 −/− and KI(Ox + ) mice. Notably, we also detected 5-carbamoylhydroxymethyluridine (nchm 5 U) and trace amounts of 5-carboxyhydroxymethyluridine (chm 5 U), the hydroxylated forms of ncm 5 U and cm 5 U, in tRNA from the MT-deficient mice (note that the R and S diastereomers of these nucleosides could not be separated chromatographically). This indicates that OxX and possibly also the ALKBH8 oxygenase will hydroxylate ncm 5 U, and to a lesser extent, cm 5 U, when mcm 5 U is absent. Enzymatic activity of recombinant ALKBH8 on murine tRNA To investigate whether the observed hypomodification of tRNA from gene-targeted mice could be reversed by recombinant enzymes, total tRNA from mouse liver was incubated with E. coli -expressed human ALKBH8, or combinations of its individual oxygenase (ALKBH8-Ox) and MT (ALKBH8-MT) domains ( Fig. 2d,e ). The results demonstrated that ALKBH8-Ox hydroxylates mcm 5 U into ( S )-mchm 5 U, and corroborated the notion that the two ALKBH8 enzymatic domains can function independently ( Fig. 2e ; see Fig. 2c for samples not treated with enzyme; Supplementary Fig. S8 ). The latter was further substantiated by the observation that the oxygenase and MT functions of ALKBH8 could be selectively inhibited by the Fe(II) chelator EDTA and the MT inhibitor S-adenosylhomocysteine, respectively ( Supplementary Fig. S8 ). Moreover, ALKBH8-Ox, but not a mutant with putative Fe(II) coordinating residues mutated, displayed the expected Fe(II)-dependent ability to convert 2OG to succinate ( Supplementary Fig. S9 ), supporting the notion that ALKBH8 is a 2OG/Fe(II) oxygenase. Modification status of from the Alkbh8-targeted mice As our results strongly indicated that is the substrate of the ALKBH8 oxygenase, we also specifically investigated the modification status of this isoacceptor from the different gene-targeted mice. WT contained not only the expected ( S )-mchm 5 U modification, but also some chm 5 U ( Fig. 2f , Supplementary Fig. S10 ), possibly due to non-enzymatic hydrolysis of the labile ester bond in ( S )-mchm 5 U, as previously reported [23] . In agreement with previous findings [22] , Alkbh8 −/− contained ncm 5 U and cm 5 U, whereas KI(Ox + ) contained nchm 5 U and chm 5 U in addition, indicating that ALKBH8-Ox, in the absence of its cognate mcm 5 U substrate can hydroxylate cm 5 U and ncm 5 U, albeit inefficiently. Moreover, KI(MT + ) displayed the expected accumulation of mcm 5 U. We performed MALDI-TOF mass spectrometry of an RNase T1 digest of the isolated , to verify its identity and to confirm the presence of mchm 5 U in its anticodon loop. Clearly, WT contained the expected ~2924.3 Da product corresponding to a ( S )-mchm 5 U-modified anticodon loop ( Figs 1d and 2g ). Moreover, from the gene-targeted mice gave rise to alternative additional peaks, agreeing with the altered modification pattern observed by LC–MS/MS. Evolutionary distribution of ALKBH8 and mchm 5 U modifications On the basis of sequence homology searches, the ALKBH8 oxygenase appears to be present in most multicellular eukaryotes, such as mammals, bee ( Apis mellifera ), worm ( Caenorhabditis elegans ) and plant ( Arabidopsis thaliana ; Supplementary Fig. S11 ). Accordingly, we detected ( S )-mchm 5 U in all these organisms ( Fig. 3a ), but neither in the budding yeast S. cerevisiae nor in the fission yeast Schizosaccharomyces pombe , which both have mcm 5 U-modified tRNAs, but lack ALKBH8. Notably, ( R )-mchm 5 U was detected only in the mammalian tissues tested (calf and mouse), and here at levels which represented ~350x the detection limit (0.003 ( R )-mchm 5 U per 10,000 unmodified nucleosides). This indicates that if ( R )-mchm 5 U is present in any of the other organisms, the level is at least two orders of magnitude lower than that in mammals. As was observed with the mcm 5 U-containing KI(MT + ) tRNA, the majority of mcm 5 U in S. cerevisiae or S. pombe tRNA could be converted to ( S )-mchm 5 U by incubation with ALKBH8-Ox ( Fig. 3b , Supplementary Fig. S12 ). Taken together, the observed activity of human ALKBH8-Ox on tRNA from distantly related organisms and the co-occurrence of ( S )-mchm 5 U and ALKBH8 suggest that hydroxylation of mcm 5 U into ( S )-mchm 5 U is performed by ALKBH8 orthologues in a wide range of eukaryotes. 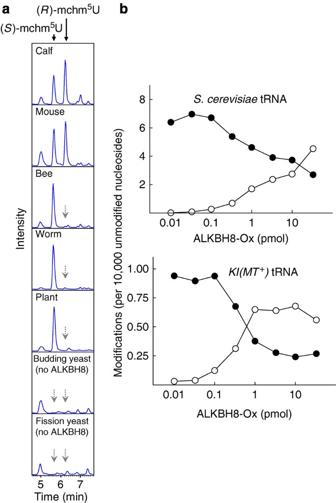Figure 3: Evolutionary conservation and cross-species activity of the ALKBH8 oxygenase. (a) mchm5U modifications in tRNA from various organisms, investigated by LC–MS/MS. (b)In vitroenzymatic activity of human ALKBH8-Ox on tRNA from the yeastS. cerevisiae(upper panel), and on tRNA from theKI(MT+) mice (lower panel). tRNA was incubated with different amounts of recombinant ALKBH8-Ox, and the levels of mcm5U (closed circles) and (S)-mchm5U (open circles) were analysed by LC–MS/MS. Figure 3: Evolutionary conservation and cross-species activity of the ALKBH8 oxygenase. ( a ) mchm 5 U modifications in tRNA from various organisms, investigated by LC–MS/MS. ( b ) In vitro enzymatic activity of human ALKBH8-Ox on tRNA from the yeast S. cerevisiae (upper panel), and on tRNA from the KI(MT + ) mice (lower panel). tRNA was incubated with different amounts of recombinant ALKBH8-Ox, and the levels of mcm 5 U (closed circles) and ( S )-mchm 5 U (open circles) were analysed by LC–MS/MS. Full size image Wobble uridine modifications and protein translation In yeast, inactivation of wobble uridine modification enzymes can impair translational decoding, as measured by decreased translation of relevant 'codon-runs' [26] , [27] . To investigate the possible effects of the extensive wobble U mis-modification observed in the Alkbh8 −/− mice, we generated reporter plasmids containing both Renilla (Rluc; internal reference) and firefly (Fluc) luciferase genes, in which Fluc, but not Rluc, translation depends on in-frame translation with a codon-run of ten identical codons ( Fig. 4a ). We generated runs of A-ending codons matching the anticodons of several tRNAs containing mcm 5 U or derivatives, and corresponding non-cognate, G-ending codon-runs as controls. We then determined the Fluc/Rluc ratio on transfection of the constructs into primary fibroblasts from Alkbh8 −/− or WT mice ( Fig. 4b ). Clearly, different A-ending codon-runs affected translation to varying degrees, but the differences between Alkbh8 −/− and WT fibroblasts were generally small, showing that the altered wobble U modification pattern of Alkbh8 −/− tRNA has a negligible effect on translation efficiency in this experimental system. 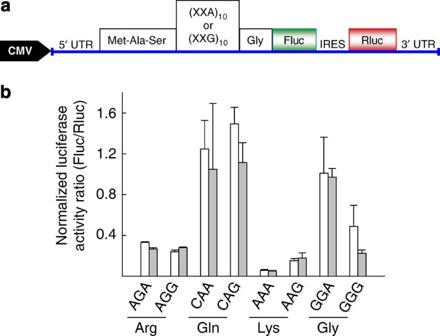Figure 4: Ability ofAlkbh8−/−tRNA to support translation. (a) Outline of the reporter construct used. The cytomegalovirus (CMV) promoter drives the expression of an mRNA (blue) encoding the protein elements indicated by boxes (drawing not to scale). (XXA)10and (XXG)10indicate runs of ten identical codons that end with A or G, respectively, and that are translated in frame with the firefly luciferase (Fluc) reporter. ARenillaluciferase (Rluc) reporter, which is translated from an internal ribosomal entry site (IRES) and independently of the codon run, serves as an internal reference. (b) Reporter constructs containing the indicated codon runs, encoding the indicated amino acids, were transfected into WT (white bars) andAlkbh8−/−(grey bars) fibroblasts. The activity of the two reporter genes was analysed and used to calculate the efficiency of translation of the codon run. Error bars indicate the standard deviation of triplicate samples. Figure 4: Ability of Alkbh8 −/− tRNA to support translation. ( a ) Outline of the reporter construct used. The cytomegalovirus (CMV) promoter drives the expression of an mRNA (blue) encoding the protein elements indicated by boxes (drawing not to scale). (XXA) 10 and (XXG) 10 indicate runs of ten identical codons that end with A or G, respectively, and that are translated in frame with the firefly luciferase (Fluc) reporter. A Renilla luciferase (Rluc) reporter, which is translated from an internal ribosomal entry site (IRES) and independently of the codon run, serves as an internal reference. ( b ) Reporter constructs containing the indicated codon runs, encoding the indicated amino acids, were transfected into WT (white bars) and Alkbh8 −/− (grey bars) fibroblasts. The activity of the two reporter genes was analysed and used to calculate the efficiency of translation of the codon run. Error bars indicate the standard deviation of triplicate samples. Full size image In this study, we have unravelled the biochemical function of the evolutionary conserved ALKBH8 oxygenase. Thus, tRNA modification is included in the broad range of reactions catalysed by 2OG/Fe(II) oxygenases, and the function of the ALKBH proteins is expanded beyond nucleic acid repair. Our data demonstrate how the MT and oxygenase activities of ALKBH8 act in a sequential manner, where the MT generates mcm 5 U, which in is further hydroxylated to ( S )-mchm 5 U by the oxygenase. Furthermore, it is demonstrated how selective inactivation of the individual domains of ALKBH8 in vivo severely distorts the modification pattern of wobble uridines, and how the ALKBH8 oxygenase, in the absence of its cognate substrate mcm 5 U, will hydroxylate ncm 5 U and cm 5 U, albeit inefficiently ( Fig. 5 ). 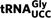Figure 5: Model for the generation of mchm5U modifications inand. The model depicts the roles of ALKBH8 and the putative oxygenase OxX in the formation of (S)-mchm5U and (R)-mchm5U inand, respectively (indicated by solid lines in arrows and borders). Dashed lines in arrows and borders indicate reactions and modifications, respectively, that occur inandwhen the ALKBH8 function is perturbed. The colour coding of borders corresponds to that of bar diagrams inFigure 2. Figure 5: Model for the generation of mchm 5 U modifications in and . The model depicts the roles of ALKBH8 and the putative oxygenase OxX in the formation of ( S )-mchm 5 U and ( R )-mchm 5 U in and , respectively (indicated by solid lines in arrows and borders). Dashed lines in arrows and borders indicate reactions and modifications, respectively, that occur in and when the ALKBH8 function is perturbed. The colour coding of borders corresponds to that of bar diagrams in Figure 2 . Full size image The present study reports the existence of two novel mammalian wobble uridine modifications, ( R )- and ( S )-mchm 5 U, and indicates that the evolution of more advanced eukaryotes has been accompanied by an increased complexity of such modifications. Most mcm 5 U-containing wobble nucleosides contain an additional, wobble restricting 2-thiolation (mcm 5 s 2 U), and the corresponding tRNAs decode in the split codon boxes. In contrast, and , which contain mchm 5 U, decode in family codon boxes. Therefore, one may speculate that the hydroxylation of mcm 5 U into mchm 5 U improves the reading of non-cognate codons; a typical feature of wobble uridine modifications found on family box tRNAs [3] , [4] . This ability may be of particular importance in higher eukaryotes, for example, mammals, which consist of a wide diversity of specialized cells, such as elongated neurons. Here, protein translation often occurs at discrete locations [28] , where low local concentrations of certain isoacceptors could necessitate the extensive use of non-cognate tRNAs in decoding. Stereoisomers are frequently formed by epimerization, and one could envision ( R )-mchm 5 U being formed by epimerization of ( S )-mchm 5 U, rather than by hydroxylation of mcm 5 U. However, our presented data strongly argue against this notion, and predict an unknown oxygenase, OxX, for generation of ( R )-mchm 5 U from mcm 5 U. First, the observation that ( R )-mchm 5 U, but not ( S )-mchm 5 U, is present in the KI(MT + ) mice indicates that the former is generated independently of the latter. Second, in the Alkbh8 −/− mice, in which the ALKBH8-Ox and ALKBH8-MT functions are both absent, total tRNA contained nchm 5 U (which is absent from WT tRNA). This presence of nchm 5 U may be explained by hydroxylation of accumulated ncm 5 U by the enzyme OxX, which normally catalyses the2 hydroxylation of mcm 5 U into ( R )-mchm 5 U. Future studies will investigate various oxygenases, including ALKBH proteins of unknown function, as candidates for the OxX function. Recently, the mammalian Tet proteins (Tet1, Tet2 and Tet3) were shown to be DNA hydroxylases converting epigenetic 5-methylcytosine (5mC) modifications into 5hmC [8] , [29] . Interesting analogies exist between ALKBH8 and the Tet proteins, as they all are 2OG/Fe(II) oxygenases acting on nucleic acids, and as they hydroxylate corresponding positions in mcm 5 U and 5mC, respectively. Conceivably, other ALKBH proteins may also catalyse reactions resulting in hydroxylation (rather than demethylation) of macromolecules. Total tRNA and isoacceptor isolation Total tRNA from S. cerevisiae and calf liver was purchased from Roche and Novagen, respectively. Total tRNA was purified from Mus musculus (liver), A. mellifera (head and thorax of worker bees), C. elegans , A. thaliana and S. pombe by using a RNA/DNA Maxi Kit (QIAGEN). Individual and isoacceptors were purified from total tRNA using 3′-biotinylated oligonucleotides ( Supplementary Table S1 ), as previously described [22] . Synthesis of mchm 5 U nucleoside standards ( R )- and ( S )-mchm 5 U were obtained by a previously reported three-step procedure [30] . The structure and homogeneity of these nucleosides derivatives were confirmed by nuclear magnetic resonance and mass spectrometry. LC–MS/MS of nucleosides The analysis was performed essentially as described [22] . Briefly, tRNA was enzymatically digested to nucleosides [31] , which were separated by reverse phase high-performance liquid chromatography on a Zorbax SB-C18 column, using a mobile phase consisting of 0.1% formic acid and a gradient of 5–50% methanol. Online mass spectrometry detection was performed using an Applied Biosystems/MDS Sciex 5000 triple-quadrupole mass spectrometer (Applied Biosystems Sciex) with TurboIonSpray probe operating in positive electrospray ionization mode. The nucleosides were monitored by multiple reaction monitoring using the nucleoside to base ion mass transitions 317.2→185.1 (mcm 5 U), 333.2→201.1 (mchm 5 U), 303.2→171.1 (cm 5 U), 319.2→187.1 (chm 5 U), 302.2→170.1 (ncm 5 U), 318.2→186.1 (nchm 5 U), 268.2→136.1 (A), 244.2→112.1 (C), 284.2→152.2 (G) and 245.2→113.1 (U). Quantification was performed by comparison with pure nucleoside standards run in between the samples. Nucleoside standards for ncm 5 U and nchm 5 U were generated from mcm 5 U and mchm 5 U as previously described [32] , whereas cm 5 U and chm 5 U were generated by mild alkaline hydrolysis of mcm 5 U and mchm 5 U (ref. 22 ). The fragmentation pattern of the nucleoside standards was in accordance with theoretical predictions, and has been included in Supplementary Figure S13 . MALDI-TOF mass spectrometry tRNA isoacceptors were digested with RNase T1 (Ambion) and samples prepared for mass spectrometry as previously described [22] . MALDI (matrix-assisted laser desorption/ionization) mass spectrometry was performed on a Perseptive Voyager STR instrument detecting positive ions in reflector TOF geometry. Spectrum processing was done with the MoverZ software (Genomic Solutions). MALDI tandem mass spectrometry was performed on a Waters QTOF Ultra MALDI instrument (Waters) with sample preparation as described above. The spectra were recorded in positive ion mode and processed with the supplied MassLynx software; additional details have been published previously [33] . Gene-targeted mice Gene-targeting strategy and screening method to verify homologous recombination are presented in Supplementary Figures S2–S5 . Expression of recombinant proteins Human ALKBH8 (aa 1–664), or its MT domain (ALKBH8-MT; aa 352–664), both in complex with human TRM112, and its AlkB domain (ALKBH8-Ox; aa 1–354) were purified as amino-terminal 6xHis-tagged protein from E. coli as previously described [22] . Enzymatic treatment of tRNA tRNA (5–10 μg) was incubated with recombinant protein (100 pmol, if not indicated otherwise) for 30 min at 37 °C in a 50 μl reaction mixture containing 25 μM S -adenosyl- L -methionine, 50 mM Tris-HCl pH 7.5, 25 mM KCl, 25 mM NH 4 Ac, 0.5 mM MgCl 2 , 2 mM ascorbic acid, 100 μM 2-oxoglutarate, 40 μM FeSO 4 , 10 U RNase inhibitor and then precipitated with 1 volume of isopropanol in the presence of 1 M NH 4 Ac and 10 μg of glycogen. Incubations with ALKBH8 and ALKBH8-MT were performed in the presence of the co-expressed and co-purified accessory protein TRM112. Pellets were washed with 70% EtOH, dried and dissolved in H 2 O. The samples were subjected to nucleoside analysis by LC–MS/MS. Codon-run reporter constructs Short dsDNA fragments containing Nco I-specific DNA overhangs at both ends and harbouring ten successive, identical Lys, Gln, Arg or Gly codons were generated by annealing oligo pairs AAA 10 -s/AAA 10 -as, AAG 10 -s/AAG 10 -as, CAA 10 -s/CAA 10 -as, CAG 10 -s/CAG 10 -as, AGA 10 -s/AGA 10 -as, AGG 10 -s/AGG 10 -as, GGA 10 -s/GGA 10 -as or GGG 10 -s/GGG 10 -as ( Supplementary Table S1 ), respectively, and inserted downstream of the translation initiation codon of the firefly luciferase gene in pDualLuc-IRES3 using its Nco I site [34] . Subsequently, Not I- Hin dIII fragments from pDualLuc-IRES3 or derivatives containing a codon-run insertion were transferred to pCMV-Script (Stratagene). Following this strategy, pDualLuc-LysAAA 10 , pDualLuc-LysAAG 10 , pDualLuc-GlnCAA 10 , pDualLuc-GlnCAG 10 , pDualLuc-ArgAGA 10 , pDualLuc-ArgAGG 10 , pDualLuc-GlyGGA 10 and pDualLuc-GlyGGG 10 were constructed ( Fig. 4a ). In vivo translation efficiency assay Primary mouse embryonic fibroblasts were maintained in DMEM (BioWhittaker) supplemented with 15% fetal bovine serum (Saveen & Werner) and 100 U per ml penicillin and streptomycin. Cells were grown to 90% confluency and transfected using a MicroPorator MP-100 (Digital Bio Technology, NanoEnTek). Cells (5×10 5 ) were transfected with pDualLuc reporter plasmids using a pulse voltage of 1,350 V, 30 ms pulse width and a 100 μl Gold Tip according to the manufacturer's instructions, and immediately after electroporation transferred to pre-warmed 12-well dishes containing DMEM without antibiotics. Cells were collected at 24 h post-transfection and the intracellular Fluc and Rluc activities were subsequently measured using a Luminometer (Turner Designs TD-20/20), using the Dual-luciferase Reporter Assay according to the manufacturer's protocol (Promega). How to cite this article: van den Born, E. et al . ALKBH8-mediated formation of a novel diastereomeric pair of wobble nucleosides in mammalian tRNA. Nat. Commun. 2:172 doi: 10.1038/ncomms1173 (2011).